Extending Noether’s theorem by quantifying the asymmetry of quantum states Noether’s theorem is a fundamental result in physics stating that every symmetry of the dynamics implies a conservation law. It is, however, deficient in several respects: for one, it is not applicable to dynamics wherein the system interacts with an environment; furthermore, even in the case where the system is isolated, if the quantum state is mixed then the Noether conservation laws do not capture all of the consequences of the symmetries. Here we address these deficiencies by introducing measures of the extent to which a quantum state breaks a symmetry. Such measures yield novel constraints on state transitions: for nonisolated systems they cannot increase, whereas for isolated systems they are conserved. We demonstrate that the problem of finding non-trivial asymmetry measures can be solved using the tools of quantum information theory. Applications include deriving model-independent bounds on the quantum noise in amplifiers and assessing quantum schemes for achieving high-precision metrology. Finding the consequences of symmetries for dynamics is a subject with broad applications in physics, from high-energy scattering experiments, through control problems in mesoscopic physics, to issues in quantum cosmology. In many cases, a complete solution of the dynamics is not possible either because it is too complex or because one lacks precise knowledge of all of the relevant parameters. In such cases, one can often still make non-trivial inferences by a consideration of the symmetries. The most prominent example is the inference from dynamical symmetries to constants of the motion in closed-system dynamics. For instance, from invariance of the laws of motion under translation in time, translation in space, and rotation, one can infer, respectively, the conservation of energy, linear momentum, and angular momentum. This result has its origin in the work of Lagrange in classical mechanics [1] , but when the symmetries of interest are differentiable, the connection is established by Noether’s theorem [2] . These days, physicists tend to use the term ‘Noether’s theorem’ to refer to the general result, and we follow this convention here. The theorem applies also in the quantum realm, where symmetries of the time evolution imply the existence of a set of observables all of whose moments are conserved [3] . The quantum case is the one of interest in this work. A symmetric evolution is one that commutes with the action of the symmetry group [4] . For instance, a rotationally invariant dynamics is such that a rotation of the state before the dynamics has the same effect as doing so after the dynamics. An asymmetry measure quantifies how much the symmetry in question is broken by a given state. More precisely, a function f from states to real numbers is an asymmetry measure [5] , [6] , [7] , [8] , [9] , [10] , [11] if the existence of symmetric dynamics taking ρ to σ implies f ( ρ )≥ f ( σ ). A measure for rotational asymmetry, for instance, is a function over states that is non-increasing under rotationally invariant dynamics. For systems interacting with an environment (open-system dynamics), where Noether’s theorem does not apply, every asymmetry measure imposes a non-trivial constraint on what state transitions are possible under the symmetric dynamics, namely that the measure evaluated on the final state be no larger than that evaluated on the initial state. For isolated systems (closed-system dynamics), the existence of a symmetric unitary for some state transition implies the existence of a symmetric unitary for the reverse transition (namely, the adjoint of the unitary); hence, each asymmetry measure is a conserved quantity under the symmetric dynamics. We show that, for transitions between mixed states, the conserved quantities one obtains in this way in general can be independent of those prescribed by Noether’s theorem. In this way, we find new conservation laws, which are not captured by Noether’s theorem. Our results also allow us to derive constraints on state transitions given discrete symmetries of the dynamics, that is, symmetries associated with finite groups, where there are no generators of the group action and it is less obvious how to apply Noether’s theorem. The inadequacy of Noether conservation laws How can we find non-trivial asymmetry measures? In the case of rotational symmetry, one might guess that the (expectation value of) components of angular momentum are good candidates. For one, a state with non-zero angular momentum is necessarily non-invariant under some rotation. For another, in closed-system dynamics, any asymmetry measure must be a constant of the motion and angular momentum certainly satisfies this condition. Nonetheless, it turns out that angular momentum is not an asymmetry measure. More generally, it turns out that none of the Noether conserved quantities, nor any functions thereof, provide non-trivial measures of asymmetry. To prove this, it is necessary to provide more precise definitions of the notions of symmetric states and symmetric time evolutions. One specifies the symmetry of interest by specifying an abstract group G of transformations and the appropriate representation thereof. For a general symmetry described by a group G , the symmetry transformation corresponding to the group element g is represented by the map ρ → g ( ρ ) where g (·)≡ U ( g )(·) U † ( g ) and U ( g ) is a unitary operator. For instance, under rotation around an axis by angle θ , the density operator of a system will be transformed as where J =( J x , J y , J z ) is the vector of angular momentum operators. A state ρ does not break the symmetry G , or is symmetric relative to group G , if for all group elements g ε G it holds that g ( ρ )= ρ . A general time evolution , which is a linear transformation from the space of density operators to itself, ρ →( ρ ), is symmetric relative to group G if it commutes with the symmetry transformation ρ → g ( ρ ) for all group elements g in group G (See Fig. 1 ). Note that this definition of a symmetric time evolution applies equally well to the cases of closed-system dynamics and open-system dynamics (see Fig. 2 ). 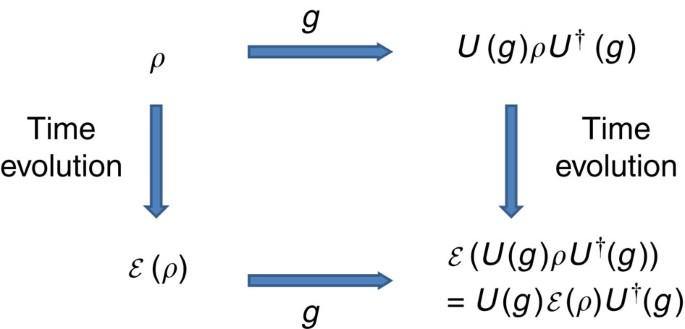Figure 1: The definition of symmetric dynamics. A time evolution is called symmetric relative to a groupGif the map describing the evolution commutes with the symmetry transformation associated with every group elementgεG. Figure 1: The definition of symmetric dynamics. A time evolution is called symmetric relative to a group G if the map describing the evolution commutes with the symmetry transformation associated with every group element g ε G . 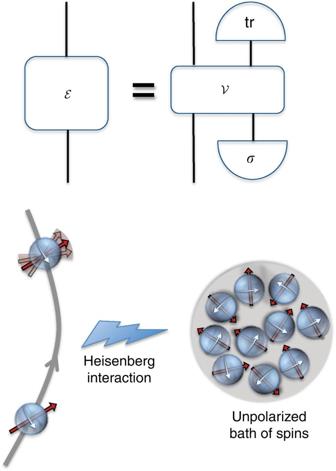Figure 2: Symmetric open-system dynamics. The top figure depicts such dynamics as a circuit. The system is coupled to an ancilla that is prepared in a symmetric stateσ, that is, [σ,U(g)]=0∀gεG, and the pair undergoes a closed-system dynamics associated with a symmetric unitary map (·)≡V·V†whereVis a unitary operator satisfying the symmetry property [V,U(g)]=0∀gεG. The overall dynamics for the system then corresponds to an open-systen dynamics associated with a completely positive trace-preserving linear map (·)≡tra[V(·⊗ρ)V†] that is symmetric, that is, (U(g)·U†(g))=U(g)(·)U†(g)∀gεG. (Here tradenotes the trace operation on the ancilla.) Furthermore, every symmetric map can be implemented in this manner31. An example of such a dynamics is a spin-1/2 system interacting via a Heisenberg spin–spin interaction (which is rotationally invariant) with a bath of spin-1/2 systems that are polarized in random directions, such that the overall state is unpolarized. This is depicted in the bottom figure. Full size image Figure 2: Symmetric open-system dynamics. The top figure depicts such dynamics as a circuit. The system is coupled to an ancilla that is prepared in a symmetric state σ , that is, [ σ , U ( g )]=0 ∀ g ε G , and the pair undergoes a closed-system dynamics associated with a symmetric unitary map (·)≡ V · V † where V is a unitary operator satisfying the symmetry property [ V , U ( g )]=0 ∀ g ε G . The overall dynamics for the system then corresponds to an open-systen dynamics associated with a completely positive trace-preserving linear map (·)≡tr a [ V (· ⊗ ρ ) V † ] that is symmetric, that is, ( U ( g )· U † ( g ))= U ( g )(·) U † ( g ) ∀ gε G . (Here tr a denotes the trace operation on the ancilla.) Furthermore, every symmetric map can be implemented in this manner [31] . An example of such a dynamics is a spin-1/2 system interacting via a Heisenberg spin–spin interaction (which is rotationally invariant) with a bath of spin-1/2 systems that are polarized in random directions, such that the overall state is unpolarized. This is depicted in the bottom figure. Full size image For a symmetry described by a Lie group G , Noether’s theorem states that every generator L of G is conserved, or equivalently, the expectation value of any function of L is conserved. Therefore, if under a unitary symmetric dynamics state ρ evolves to state σ , then all the implications of Noether’s theorem for quantum theory can be summarized as: for every generator L of G . We can now make precise the sense in which Noether-conserved quantities yield no non-trivial measures of asymmetry: for a symmetry corresponding to any compact Lie group G , any asymmetry measure f that is a continuous function of only the Noether-conserved quantities is trivial, that is, it takes the same value for all states. The proof is provided in the Methods section, but we will here sketch the main idea. States that are asymmetric must necessarily fail to commute with some generator of the group, say L , and consequently must have coherence between different eigenspaces of L (for example, a state that is non-invariant under phase shifts necessarily has coherence between eigenspaces of the corresponding number operator). A non-trivial asymmetry measure must be able to detect such coherence. If the state were known to be pure, then the presence of such coherences would be revealed by a non-zero variance over L . However, an asymmetry measure is a function over all states, and there exists mixed states that have non-trivial variance over L , even though they have no coherence between the eigenspaces of L . Hence, the value of the second moment of L has no information about the asymmetry properties of the state. By the same logic, no moment of L has any information about the asymmetry properties of the state. It follows that the problem of devising measures of asymmetry is non-trivial. Nonetheless, it can be solved by taking an information-theoretic perspective on symmetric dynamics. Measures of asymmetry from measures of information Consider the problem of communicating information about a direction in space (See Fig. 3 ). It is clear that to be able to succeed in this task, one needs to use states that break the rotational symmetry. Furthermore, intuitively we expect that to transfer more directional information one needs to use states that are more asymmetric. This suggests that one can quantify rotational asymmetry by the amount of information a state encodes about orientation. 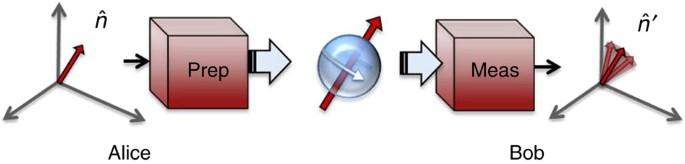Figure 3: Quantum communication protocol for sending information about direction. Alice chooses a directionand prepares a spin-jsystem in the coherent state in this direction, that is, she prepares the statewhere. Then she sends this spin system to Bob. Bob performs a measurement on the system and obtains an estimate of, denoted. The uncertainty principle implies that there is a fundamental limit on the accuracy of Bob’s estimate which is determined byj: the variance of the estimated angles are bounded by a constant factor times 1/j2. Within the set of coherent states, therefore, the amount of directional information, and hence the rotational asymmetry, increases withj. Figure 3: Quantum communication protocol for sending information about direction. Alice chooses a direction and prepares a spin- j system in the coherent state in this direction, that is, she prepares the state where . Then she sends this spin system to Bob. Bob performs a measurement on the system and obtains an estimate of , denoted . The uncertainty principle implies that there is a fundamental limit on the accuracy of Bob’s estimate which is determined by j : the variance of the estimated angles are bounded by a constant factor times 1/ j 2 . Within the set of coherent states, therefore, the amount of directional information, and hence the rotational asymmetry, increases with j . Full size image To make this connection precise, we note that if ρ → σ by some symmetric dynamics then by definition this dynamics also takes every state in the group orbit of ρ to the corresponding state in the group orbit of σ , that is, g ( ρ )→ g ( σ ) for all g ε G . The set of states { g ( ρ ) : g ε G } can be understood as a quantum encoding of a classical variable that ranges over the elements of the group G , and the dynamical evolution realizing g ( ρ )→ g ( σ ) for all g ε G can be understood as a kind of data processing. From the existence of such a data processing, it follows that the σ -based encoding must contain no more information about g than the ρ -based encoding. A measure of the information content of an encoding is a function from encodings to reals that is nonincreasing under data processing. Specifically, I is a measure of information if for any two different quantum encodings of a classical random variable x ε X , { ρ x : x ε X } and { σ x : x ε X }, the existence of a dynamical evolution that maps ρ x to σ x for all x ε X implies that I ({ ρ x : x ε X })≥ I ({ σ x : x ε X }). (In the context of information theory, the monotonicity of a measure of information is known as the data processing inequality.) It follows that if we define a real function f such that its value on a state is the measure of information I of the group orbit of that state, that is, f ( ρ ) ≡ I ({ g ( ρ ) : g εG}), then f is a measure of asymmetry. The proof is simply that if ρ is mapped to σ by some symmetric dynamics, then for all g ε G the state g ( ρ ) is mapped to g ( σ ) by that dynamics, and consequently I ({ g ( ρ ) : g ε G })≥ I ( g ( σ ) : g ε G ), which implies f ( ρ )≥ f ( σ ). Quantum information theorists have defined many measures of information and for each of these we can obtain a measure of asymmetry. We mention a few that can be derived in this manner (details of the derivation are provided in the Methods section). Let p ( g ) be an arbitrary probability density over the group manifold, and define the twirling operation weighted by p ( g ) as p ≡∫ dg p ( g ) g . Let S ( ρ ) ≡ −tr( ρ log ρ ) be the von Neumann entropy. The function is an asymmetry measure. We will refer to such a measure as a Holevo asymmetry measure. The intuition behind it is as follows: if a state is close to symmetric, then it is close to invariant under rotations and mixing over all rotations does not change its entropy much, while, if it is highly asymmetric, then under rotations it covers a broader manifold of states and hence mixing over all rotations increases the entropy significantly. Let the matrix commutator of A and B be denoted by [ A , B ] and the trace norm (or ℓ 1 -norm) by . For any generator L of the group action, the function is a measure of asymmetry. This measure formalizes the intuition that the asymmetry of a state can be quantified by the extent to which it fails to commute with the generators of the symmetry. For any generator L , and for 0< s <1, the function is a measure of asymmetry. This quantity was introduced by Wigner and Yanase [12] with s =1/2 and generalized by Dyson to arbitrary s . While it has attracted much interest, its monotonicity under symmetric dynamics—and hence its interpretation as a measure of asymmetry—was not previously recognized. For all of these examples, if ρ is a symmetric state then the asymmetry measure has value zero. Furthermore, for F L and S L,s , if ρ is a pure state then the measure reduces to the variance over L . The measures F L and S L,s can both be understood as quantifying the ‘coherent spread’ over the eigenvalues of L . As discussed earlier, this is precisely what the variance over L (or any function of L ) could not do. Inadequacy of Noether conservation laws for isolated systems We have seen how conservation of all the Noether quantities is neither a necessary nor a sufficient condition for the possibility of a state transition in open-system symmetric dynamics. We now turn to closed-system dynamics. Recalling that measures of asymmetry are conserved quantitites in closed-system symmetric dynamics and that any non-trivial measure of asymmetry cannot be expressed as a function of the Noether quantities alone, one is led to expect that the constraints obtained from the conservation of non-trivial measures of asymmetry can be independent of the constraints obtained from Noether conservation laws. In this section, we show that this is indeed the case. Although Noether conservation laws provide necessary conditions for a state transition to be achievable in a closed-system symmetric dynamics, they do not provide sufficient conditions. Necessity follows from the fact that if there exists a unitary U such that σ = U ρ U † and having the relevant symmetry (that is, [ U , L ] for every generator L of G ), then the Noether conditions (Equation 1) are satisfied. Insufficiency is established by the following counterexample, which exhibits a state transition that does not violate any Noether conservation law, but that violates the conservation law for a non-trivial measure of asymmetry. Consider a spin-1/2 system that also has some other independent degree of freedom, which is invariant under rotation, denoted by the observable Q . Let denote eigenstates of spin along the -axis, and let | q 1 ›, | q 2 › denote orthogonal eigenstates of Q . Then define and We can easily check that: (1) the state transition ρ → σ is impossible by rotationally symmetric closed-system dynamics (but possible by dynamics that break rotational symmetry, namely, a rotation around by π/2, so that the transition would not be forbidden were it not for considerations of symmetry). (2) All constraints implied by Noether’s theorem hold, that is, the conditions of Equation (1) for generators of rotations are satisfied, and therefore Noether’s theorem does not forbid this transition. Condition (2) is straightforward to verify. The truth of (1) can be made intuitive by noting that ρ is symmetric under rotations about the -axis while σ is not, such that a transition from ρ to σ is symmetry breaking and hence impossible by rotationally symmetric dynamics. One can derive this same conclusion using asymmetry measures. Consider the Holevo asymmetry measure Γ p for the probability density p that is vanishing for all rotations besides those about the axis, where it assigns a uniform measure over all angles φ ε[0, 2π]. (More precisely, if Ω , φ denotes the element of SO(3) corresponding to a rotation by φ about the axis and dΩ denotes the uniform measure over SO(3), then the probability density p is defined as follows: for any arbitrary function f over SO(3), ). One easily verifies that Γ p ( ρ )=0 and Γ p ( σ )=1, that is, Γ p increases in this state transition, thereby demonstrating that it cannot be achieved by rotationally symmetric dynamics. We have shown that constants of the motion derived from asymmetry measures can capture restrictions on the dynamics that are not captured by Noether’s theorem. Special case of closed-system dynamics of pure states One final special case remains to be considered. Might it be that conservation of the Noether-conserved quantities is the necessary and sufficient condition for the possibility of state interconversion under symmetric closed-system dynamics when the states are pure? In this case, the answer is yes. It has previously been shown [13] that the asymmetry properties of a pure state | ψ › are completely determined by the complex function ‹ ψ | U ( g )| ψ › over the group manifold, called the characteristic function. Equality of characteristic functions is the necessary and sufficient condition for two pure states to be reversibly interconvertible under symmetric unitary dynamics [13] . Expanding U ( g ) in a power series over the generators, one deduces that for connected compact Lie groups, such as the group of rotations, the equality of all moments of the generators is equivalent to the equality of the characteristic functions. Consequently, for pure states undergoing reversible dynamics with such a symmetry, Noether’s theorem, that is, Equation (1), captures all of the consequences of the symmetry. In practice, we are always faced with some loss of information under any quantum dynamics, due to the ubiquity of decoherence, and there is always some noise in our preparation of the initial state. Therefore, reversible dynamics of pure states is an idealization that is never achieved in practice, and as soon as one departs from it Noether’s theorem is inadequate for describing the consequences of symmetry. Applications of measures of asymmetry Phase-insensitive quantum amplifiers are examples of open-system dynamics that have a symmetry property. Consequently, from the nonincrease of measures of asymmetry, we can derive bounds on their performance. The purpose of a quantum amplifier is to increase the expectation value of some observable, such as the number operator for optical fields [14] . In most studies, constraints on amplification are obtained for specific physical models of the amplifier. Furthermore, the analysis is typically done separately for linear and nonlinear amplifiers as well as for deterministic and nondeterministic amplifiers [15] . By contrast, the constraints that can be found with our techniques follow from assumptions of symmetry alone. For instance, in optics they follow from the fact that the amplifier is phase-insensitive. They are therefore model independent and can be applied whether the amplifier is linear or nonlinear, deterministic or nondeterministic. Here is an example of such a constraint, arising from the Holevo measure of asymmetry. If ρ is mapped to σ by a symmetric amplifier, then which asserts that the change in entropy under the transition has a non-trivial lower bound. For instance, suppose that ρ is a state of a spin-1/2 system, while σ is a state of a spin- j system for j >>1/2. Suppose further that the probability density p in p is chosen to be the uniform measure over the symmetry group (which in this problem is SO(3)), so that S ( p ( ρ ))=1 while S p ( σ )) is large (logarithmic in j ). The inequality then implies that S ( ρ )− S ( σ ) must be large. This demonstrates that in the case of rotationally symmetric open-system dynamics, an increase in the value of the angular momentum along some axis is not prohibited as long as entropy increases. This ensures that the distinguishability of states at the output is not more than the distinguishability of states at the input, so that the information content has not increased (see Fig. 4 ). 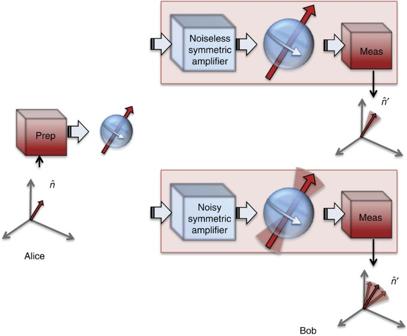Figure 4: An example of information-theoretic constraints on state transitions in symmetric open-system dynamics. Suppose that there were a rotationally symmetric open-system dynamics which transforms the coherent state aligned in the-direction,, to the coherent statewhere, that is, a rotationally symmetric noiseless amplifier. If this were possible then in the communication protocol described inFig. 3, Bob could first apply this dynamics and then estimate the directionusing the state. Such a strategy would yield an estimate with variance proportional to, which is better than what is allowed by the fundamental quantum limit. Hence, we conclude that the state transition is not possible by rotationally symmetric dynamics. In contrast, for a similar rotationally symmetric dynamics, which adds noise to the state, such thatis not mapped tobut to a mixed spin-state, as long as the noise is large enough to ensure that Bob can only estimatewith a variance proportional to, considerations of information content do not rule out the transition. Indeed, one can always increase the expectation value of the angular momentum if there is a compensating increase in the entropy. Figure 4: An example of information-theoretic constraints on state transitions in symmetric open-system dynamics. Suppose that there were a rotationally symmetric open-system dynamics which transforms the coherent state aligned in the -direction, , to the coherent state where , that is, a rotationally symmetric noiseless amplifier. If this were possible then in the communication protocol described in Fig. 3 , Bob could first apply this dynamics and then estimate the direction using the state . Such a strategy would yield an estimate with variance proportional to , which is better than what is allowed by the fundamental quantum limit. Hence, we conclude that the state transition is not possible by rotationally symmetric dynamics. In contrast, for a similar rotationally symmetric dynamics, which adds noise to the state, such that is not mapped to but to a mixed spin- state, as long as the noise is large enough to ensure that Bob can only estimate with a variance proportional to , considerations of information content do not rule out the transition. Indeed, one can always increase the expectation value of the angular momentum if there is a compensating increase in the entropy. Full size image A second application of measures of asymmetry is to quantify quantum coherence [16] , [17] . Coherence is at the heart of many distinctly quantum phenomena from interference of individual quanta to superconductivity and superfluidity. On the practical side, coherence is the property of quantum states that is critical for quantum phase estimation: a coherent superposition of number eigenstates, such as , is sensitive to phase shifts, while an incoherent mixture, such as , is not. Phase shifts, however, are symmetry transformations. Therefore, states with coherence are precisely those that are asymmetric relative to the group of phase shifts. It follows that we can define a measure of coherence as any function that is nonincreasing under phase-insensitive time evolutions [8] . Hence the measures of asymmetry proposed here—Equations (2), (3) and (4)—can be used as measures of coherence relative to the eigenspaces of the generator L (that is, as the ‘coherent spread’). Finally, measures of asymmetry are important because asymmetry is the resource that powers quantum metrology (this contrasts with the more standard view that the relevant resource is entanglement, although sometimes measures of entanglement may be related to measures of asymmetry). Metrology involves estimating a symmetry transformation [18] . In the general case, the set of symmetry transformations forms a non-Abelian group, such as the group of rotations, but, in the most common example, it is the Abelian group of phase shifts (in which case asymmetry corresponds to coherence). We focus on this example to illustrate the idea. To estimate an unknown phase shift φ of an optical mode, one prepares the mode in the state ρ , subjects it to the unknown phase shift, leaving it in the state e i φ N ρe − i φ N , where N is the number operator, and finally one measures it. The usefulness of a particular state ρ can be quantified by any measure of the information content of the ensemble { e i φ N ρe − i φ N : φ ε[0, 2π]}, but, as shown above, every such measure is a measure of the asymmetry of ρ relative to phase shifts. The figure of merit for a metrology task is therefore a measure of asymmetry and dictates the optimal ρ . Suppose, for instance, that one seeks an unbiased estimator of φ and the figure of merit is the variance in , denoted . It has previously been shown [19] that for a state ρ , we have (a quantum generalization of the Cramer-Rao bound) where is the Wigner-Araki-Dyson skew information of order s =1/2, defined in Equation (4). Hence, it is the latter measure of asymmetry that is relevant in this case. To date, the field of quantum information theory has been primarily concerned with problems that are of interest to computer scientists. It has become apparent, however, that there are also important applications to problems that are of interest to physicists, such as simulating many-body systems [20] , [21] , [22] ; describing quantum phase transitions and topological order [23] , [24] , [25] ; and understanding black hole thermodynamics [26] . We have here presented another example of this broadening of the field’s scope by demonstrating its applicability to a prominent and generic physics problem, that of deducing the consequences of symmetries for the evolution of dynamical systems. Specifically, we have demonstrated a duality between state evolution under constrained dynamics and evolution of a set of states (a quantum encoding of information) under unconstrained dynamics. This duality has been used to build measures of the extent to which a quantum state breaks a symmetry from measures of the extent to which it can encode information about a classical variable that ranges over the elements of the symmetry group. In symmetric open-system dynamics, where Noether’s theorem does not apply, the monotonicity of such measures of asymmetry yields non-trivial constraints on state transitions. These can be understood as analogues of the monotonicity of the entropy under thermodynamically cyclic processes, the standard expression of the second law of thermodynamics. In symmetric closed-system dynamics, one also obtains new results: for every non-trivial measure of asymmetry, there are state transitions under closed-system dynamics that are not forbidden by the traditional Noether conservation laws, but are forbidden by the new conservation law for that measure. Our analysis prompts the question: what are the necessary and sufficient conditions on two quantum states (not both pure) for it to be possible to map one to the other under symmetric dynamics? Such conditions would capture all of the consequences of the symmetry of the dynamics. The question remains open but our results suggest that adopting an information-theoretic perspective may be the most expedient path to a solution. Noether conserved quantities cannot specify the asymmetry We here prove that for symmetries corresponding to compact Lie groups, functions of Noether-conserved quantities yield only trivial measures of asymmetry. In the case of finite groups, there are no generators of the group action, and therefore we cannot generate Noether-conserved quantities in the standard way. Nonetheless, we can show that a similar result holds in this case as well. We phrase our general result (which applies to both compact Lie groups and finite groups) in terms of characteristic functions. Recall that the characteristic function of a state ρ is the expectation value of the unitary representation of the group, tr( ρU ( g )), which is a complex function over the group manifold. Then we can prove the following theorem about measures of asymmetry. Theorem 1: let f be an asymmetry measure for a finite or compact Lie group G with unitary representation U . Assume that f depends on the characteristic function of the state alone, that is, for some functional . Furthermore, in the case of compact Lie groups, assume that f is continuous. Then f ( ρ ) is independent of ρ , hence f is a trivial measure of asymmetry. In the case of compact Lie groups, the characteristic function of a state ρ uniquely specifies all the moments tr( ρ L k ) for all generators L of the symmetry; this can be seen by considering the Taylor expansion of U ( g ) around the identity. Therefore, the theorem implies that if a continuous measure of asymmetry can be expressed entirely in terms of the Noether-conserved quantities alone, that is, in terms of moments of the form tr( ρL k ), then it should be a constant function independent of ρ . Proof of theorem 1 : we first present the proof for the case of finite groups and then we explain how the result can be generalized to the case of compact Lie groups as well. Suppose * is the Hilbert space of a physical system on which the unitary representation g → U ( g ) of the symmetry group G acts as the left regular representation, that is, * has an orthonormal basis denoted by {| g ›: g ε G } such that It turns out that on this space we can define another representation of G , called the right regular representation denoted by g → V R ( g ), such that Then one can easily see that these two representations of G on * commute, Define to be the quantum operation that averages over all symmetry transformations, ≡∑ g ε G g . Let e ε G be the identity element of the group. We have where to get the last equality we have used the fact that the two representations commute, Equation (10). Hence, the characteristic function of the state | e ›‹ e | is equal to the characteristic function of the state (| e ›‹ e |). This means that for any measure f whose value for a given state depends only on the characteristic function of that state, we have As we have seen before, however, for any asymmetry measure, the value of the measure is the same for all symmetric states and furthermore this value is the minimum value of that function over all states. Given that (| e ›‹ e |) is a symmetric state, it follows that Now consider an arbitrary state ρ on a Hilbert space where the projective unitary representation of the symmetry group G is g → T ( g ). Then, one can easily show that there exists symmetric quantum channels that map the state | e ›‹ e | on * to the state ρ on . One such channel is described by the map However, the fact that ρ is symmetric together with the fact that f is an asymmetry measure implies that for any state ρ it holds that This together with (Equation 12) implies that for an arbitrary state ρ , and so the asymmetry measure f is constant over all states. This completes the proof for the case of finite groups. In the following, we prove that making the extra assumption that the asymmetry measure is also continuous, this result can be extended to the case of compact Lie groups. Note that in this case the regular representation of the group is not finite dimensional. Nonetheless, as has been noted previously [4] , [27] , there still exists a sequence of finite d-dimensional spaces, { d : d ε }, and for each d an over-complete basis {| g ›: g ε G } such that the unitary representation g → U ( g ) of the symmetry group G acts as Furthermore, for a given pair of distinct group elements, g 1 ≠ g 2 , one can make the inner product ‹ g 2 | g 1 › arbitrarily close to zero in the limit of large d [4] , [27] . In this limit, the state | e ›‹ e | has the maximal asymmetry in the sense that for any given state ρ on an arbitrary Hilbert space , there exists a symmetric channel ρ such that The symmetric channel ρ can be defined in a manner similar to how it was defined for the case of finite groups, namely, We can also define another representation of G on d , denoted g → V R ( g ), such that Then one can easily see that these two representations of G on d commute, Therefore, using the same argument that we used for the case of finite groups, we can prove that tr(| e ›‹ e | U ( g ))=tr((| e ›‹ e |) U ( g )) where e is the identity element of the group G . Therefore, for any measure f whose value for a given state depends only on the characteristic function of that state, it holds that Furthermore, because f is an asymmetry measure and because ρ is a symmetric channel, we have The above two equations imply that Given that f is assumed to be continuous, Equation (17) implies that This, together with Equation (23), proves that for any arbitrary state ρ in an arbitrary finite dimensional space , it holds that Therefore, in the case of compact Lie groups, any continuous asymmetry measure which only depends on the characteristic function of the state is a constant function. This completes the proof. Derivation of some families of asymmetry measures We now apply the recipe described in the Results section to generate various measures of asymmetry from measures of information. Specifically we prove that the functions Γ p , F L and S L,s , defined in Equations (2), (3) and (4) respectively, are indeed measures of asymmetry, and we say a bit more about their properties. Along the way, we derive some other families of asymmetry measures. Our first example starts from a family of information measures that are based on the Holevo quantity [28] . For a set of states { ρ x : x ε X }, and a probability distribution p x over X , the Holevo quantity is defined as where S ( ρ )≡ −tr( ρ log ρ ) is the von Neumann entropy of the state ρ (if x is a continuous variable, and p ( x ) is a probability density, we simply replace sums by integrals). It is well known that this quantity is non-increasing under data processing, hence it is a measure of information [28] . Taking the classical variable x ε X to be the variable g ε G (which ranges over the elements of the relevant group), and using the argument provided in the Results section, the Holevo quantity yields a family of asymmetry measures, one for every probability density p ( g ) over the group manifold (probability distribution for the case of a finite group). Specifically, it yields Γ p ( ρ )≡ S ( p ( ρ ))− S ( ρ ) (previously defined in Equation (2)), where p ≡∫ dg p ( g ) g is the superoperator that performs a p -weighted average over the group action. This justifies the claim from the Results section that Γ p is an asymmetry measure and explains why it is appropriate to call it a Holevo asymmetry measure. Note that for any symmetric state ρ and any arbitrary probability distribution p ( g ), Γ p ( ρ )=0. Also, note that for any probability distribution p ( g ) which is non-zero for all G , and for any state that breaks the symmetry, Γ p ( ρ )≠0. For the special case of a uniform weighting, this measure has been proposed previously [7] and proven to be monotonic under symmetric operations using a different type of argument. The rest of the families of asymmetry measures we consider are derived from a particular subclass of measures of the information content of a set of quantum states: those that consider the distinguishability of just a single pair of states within the set. A measure of distinguishability is defined to be a function D from pairs of states to the reals, such that for any pair of states ρ 1 and ρ 2 and any quantum channel , Specializing to the case of interest here, where the state provides information about the variable g ε G , we focus on the distinguishability of two elements in the group orbit of ρ . Without loss of generality, we can choose the pair to be ρ and g ( ρ ) for some g ε G . Consider a Lie group G . Take the distinguishability measure to be the trace distance, where is the trace norm (or ℓ 1 -norm) of the operator A . It is well known that the trace distance satisfies Equation (26) and hence constitutes a measure of the distinguishability of a pair of states [29] . Therefore, we can define an asymmetry measure using this distinguishability measure, namely, This family of measures, based on the trace norm, supplements those that were discussed in the Results section. The latter are derived as follows. Since G is a Lie group, we can consider group elements g ε G that are infinitessimally close to the identity element. Specifically, we can consider U ( g )= e i θ L for some generator L and phase θ , and in the limit where θ →0, we have Hence, we conclude that for any generator L of the Lie group the function F L ( ρ )≡||[ ρ , L ]|| 1 (previously defined in Equation (3)) is an asymmetry measure. Any state ρ that is symmetric (that is, invariant under the group action) necessarily commutes with all the generators of the group action, so for such states, F L ( ρ )=0 for all L . More generally, a state ρ is invariant under the subgroup of G that is generated by L if and only if F L ( ρ )=0. In other words, state ρ can only be asymmetric relative to this subgroup if it has some coherence over the eigenspaces of L , that is, if [ ρ , L ]≠0. Therefore, in retrospect one would naturally expect that some operator norm of the commutator [ ρ , L ] should be a measure of asymmetry relative to this subgroup. This intuition does not, however, tell us which operator norm to use. Our result shows that the trace norm does the job. The asymmetry measure F L also reduces to a simple expression for pure states: it is proportional to the square root of the variance of the observable L , that is, Given that a superposition over the eigenspaces of L that is totally incoherent (that is, a mixture over the eigenspaces) has vanishing asymmetry according to this measure, while a superposition over these eigenspaces that is totally coherent has asymmetry that depends only on the variance over L , this asymmetry measure seems to succeed in quantifying the amount of variance over L that is coherent, which one might call the ‘coherent spread’ over the eigenspaces of L . We turn to our third and final example of a family of asymmetry measures. We take as our measure of distinguishability the relative Renyi entropy of order s , defined as For s ε(0, 1), it is well known that D s satisfies Equation (26) and is therefore a valid measure of distinguishability [30] . It follows that is an asymmetry measure, one that we we did not discuss in the Results section. As in the previous example, by considering D s ( ρ , g ( ρ )) for group elements that are infinitessimally close to the identity element, we can derive a measure of asymmetry for any arbitrary generator L of the group. Using this argument, we can show that for any s ε(0, 1) and any generator L , the function S L,s ( ρ )≡tr( ρL 2 )−tr( ρ s Lρ (1− s ) L ) (previously defined in Equation (4)) is a measure of asymmetry. The family of measures of the form of S L,s have been previously studied under the name of the Wigner-Yanase-Dyson skew information [12] , but their status as measures of asymmetry had not been recognized. If ρ is a symmetric state, then it commutes with all generators of the group, and so S L,s ( ρ )=0. We also find this measure to be zero when ρ is not symmetric, but is invariant under the subgroup of G generated by L . For pure states, this measure reduces to the variance of the observable L , that is, Again, we see that a mixture over the eigenspaces of L has vanishing S L,s , while a coherent superposition over these eigenspaces has S L,s equal to the variance over L . Consequently, just as we found for F L , the asymmetry measure S L,s can be said to quantify the coherent spread over the eigenspaces of L . How to cite this article: Marvian, I. & Spekkens, R. W. Extending Noether’s theorem by quantifying the asymmetry of quantum states. Nat. Commun. 5:3821 doi: 10.1038/ncomms4821 (2014).